Localizing internal friction along the reaction coordinate of protein folding by combining ensemble and single-molecule fluorescence spectroscopy Theory, simulations and experimental results have suggested an important role of internal friction in the kinetics of protein folding. Recent experiments on spectrin domains provided the first evidence for a pronounced contribution of internal friction in proteins that fold on the millisecond timescale. However, it has remained unclear how this contribution is distributed along the reaction and what influence it has on the folding dynamics. Here we use a combination of single-molecule Förster resonance energy transfer, nanosecond fluorescence correlation spectroscopy, microfluidic mixing and denaturant- and viscosity-dependent protein-folding kinetics to probe internal friction in the unfolded state and at the early and late transition states of slow- and fast-folding spectrin domains. We find that the internal friction affecting the folding rates of spectrin domains is highly localized to the early transition state, suggesting an important role of rather specific interactions in the rate-limiting conformational changes. In spite of the complexity of protein folding, which involves the interactions of thousands of atoms, the experimentally observed kinetics of folding can often be described in terms of simple activated reactions that lead to the interconversion between well-defined thermodynamic states. However, experiments have recently started to reveal more of the kinetic complexity underlying the folding process. Examples are the identification of the relaxation dynamics of ‘downhill’ folding [1] , [2] , the measurement of transition path times [3] or the presence of internal friction [4] , [5] , [6] , [7] , [8] . These observations can no longer be accounted for by simple chemical kinetics, but require more detailed physical concepts; in this way, they provide an important link to current theories of protein folding [9] , [10] , [11] , [12] and molecular simulations [13] , [14] . A topic that is attracting increasing interest is the role of internal friction in the folding process. The experimental identification of internal friction is commonly based on a deviation from the direct proportionality of the folding time (the inverse folding rate coefficient) to solvent viscosity, resulting in a non-zero value of the folding time when extrapolated to a solvent viscosity of zero [5] . This observation indicates that the folding (or unfolding) rate is not only influenced by friction caused by collisions with solvent molecules (solvent or ‘external’ viscosity) but also by friction within or between parts of the protein [15] (protein or ‘internal’ viscosity). The molecular cause of internal friction is often difficult to identify in detail, but in principle, it can originate from any mechanism that leads to a dissipation of energy into internal degrees of freedom of the protein that do not contribute to progress along the folding reaction. Such mechanisms could range from random collisions with surrounding protein atoms to dihedral angle rotations or the transient formation and breakage of side chain or backbone interactions [5] , [16] , [17] . We use the term ‘internal friction’ to distinguish it from effects on the dynamics that scale with the bulk solvent viscosity and from activation energy terms. Based on recent experimental results, it has been suggested that internal friction effects can be particularly obvious for the kinetics of very fast-folding proteins, where the timescales characterizing the crossing of the transition state region (and even the unfolded state dynamics) can be slow enough to significantly affect the progress of the folding reaction [4] , [6] . For slower-folding proteins, however, such effects have largely remained undetectable [5] , [18] , [19] , [20] , [21] . It thus came as a surprise when recent experiments provided evidence for pronounced internal friction in the rate-limiting transition state for folding of two spectrin domains [8] . Although the folding time of the fast-folding spectrin domain R15 is directly proportional to solvent viscosity, as observed previously for other millisecond folders [18] , [19] , [20] , [21] , the folding of the structurally very similar domains R16 and R17 is much slower, and the solvent viscosity dependence of their folding times is dramatically reduced. Wensley et al . [8] concluded that the slow folding of R16 and R17 is at least in part due to internal friction. However, it has remained unclear whether this unusually large contribution of internal friction in R16 and R17 is present throughout the energy landscape underlying the folding reaction or whether it is confined to the transition state region. The role of internal friction in protein folding is of great interest also for the theoretical description of protein folding. A model that is frequently used to conceptualize protein-folding dynamics, especially for the analysis of simulations and experiments, is that of diffusion on a free energy surface [3] , [7] , [9] , [22] , [23] , [24] , [25] , [26] . In the simplest case, the folding dynamics are represented in terms of diffusion along a single reaction coordinate. Even though the required projection of the large number of degrees of freedom bears the risk of obscuring structural or mechanistic details [10] , [25] , suitable reaction coordinates that lead to a faithful description of the folding kinetics and mechanisms can often be identified [16] , [24] , [25] . However, the effective diffusion coefficient can then no longer be assumed to be invariant along the resulting free energy surface [16] , that is, as the polypeptide chain transits from the highly disordered unfolded state via its transition state ensemble towards the natively folded structure. Conceptually, diffusive models thus allow effects on protein-folding dynamics to be partitioned into differences in barrier heights on the one hand and differences in effective diffusion coefficients on the other [16] , [24] , [26] , [27] , [28] (even though this partitioning will depend on the choice of the reaction coordinate and can thus be somewhat ambiguous). The internal friction observed experimentally is expected to affect the diffusion coefficient, and therefore provides an opportunity to address the question of the position dependence of the diffusion coefficient along the folding reaction. Here we assess internal friction in the spectrin domains with two complementary approaches. The first is single-molecule Förster resonance energy transfer (FRET) combined with nanosecond fluorescence correlation spectroscopy (nsFCS), which can be used to quantify unfolded state dynamics down to the nanosecond range [29] , [30] . The second approach is the analysis of denaturant-dependent protein-folding kinetics, which allows us to differentiate the viscosity dependencies of the folding and unfolding rates over the early and late transition states of the slow folders R16 and R17 [31] , [32] . By quantitatively comparing the contributions of internal friction to the dynamics in (a) the compact unfolded state, (b) the early transition state and (c) the late transition state, we can establish whether the internal friction is evenly distributed or localized to specific regions along the free energy surface. Single-molecule FRET experiments In our single-molecule analysis, we focus on R15 and R17, the domains showing the lowest and the highest contributions of internal friction to their folding kinetics, respectively [8] . To investigate the spectrin domains with single-molecule FRET, variants of R15 and R17 with two cysteine residues were prepared and labelled with Alexa 488 and 594 as FRET donor and acceptor, respectively ( Fig. 1a ). Single-molecule FRET by confocal detection of freely diffusing molecules allows the separation of folded and unfolded subpopulations in transfer efficiency histograms ( Fig. 1b ), and thus the investigation of unfolded state properties even in the presence of a majority of folded molecules. As expected from previous observations on other proteins [33] , [34] , unfolded spectrin domains undergo a continuous compaction when the denaturant concentration is reduced and native conditions are approached (see Fig. 1c ). The transfer efficiencies and fluorescence lifetimes ( Supplementary Fig. S1 ) of the unfolded subpopulation can be used to quantify the dimensions of the unfolded state based on the intramolecular distance distributions of simple polymer models [33] , [35] , [36] , [37] , [38] , [39] . In a second step, the dynamics of the unfolded polypeptide are described in terms of diffusion on the potential of mean force corresponding to this distance distribution. To determine the relaxation time of the system (that is, the reconfiguration time, τ r , of the chain), we use nsFCS [29] , [30] , [40] (see Supplementary Information for details), which reports directly on the timescale of the distance fluctuations between the donor and acceptor chromophores ( Fig. 1d–f ). 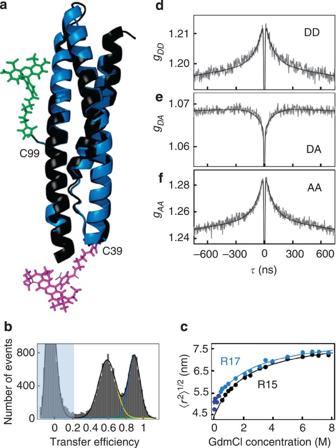Figure 1: Single-molecule spectroscopy of spectrin domains. (a) Superposition of structural representations of R15 (black) and R17 (blue) with donor (green) and acceptor (magenta) dyes at positions 39 and 99 (note that labeling is not specific). (b) Representative FRET efficiency histogram of R15 39-99 in 1.0 M GdmCl, with fits to the native and unfolded subpopulations at high- and low-transfer efficiency, respectively. The peak in the shaded range corresponds to molecules without an active acceptor fluorophore. (c) Root mean squared end-to-end distance,r21/2, of the 39-99 segments of R15 (black) and R17 (blue) calculated from the unfolded state transfer efficiencies. (d–f) Representative nanosecond fluorescence correlations of donor–donor (gDD,d), donor–acceptor (gDA,e) and acceptor–acceptor (gAA,f) fluorescence intensities for R15 at 1.2 M GdmCl. The set of DD, DA and AA correlations for each variant and GdmCl concentration are fitted globally with a common decay rate on the 100-ns timescale, which reports on the reconfiguration of the unfolded chain (for details, seeMethods). Figure 1: Single-molecule spectroscopy of spectrin domains. ( a ) Superposition of structural representations of R15 (black) and R17 (blue) with donor (green) and acceptor (magenta) dyes at positions 39 and 99 (note that labeling is not specific). ( b ) Representative FRET efficiency histogram of R15 39-99 in 1.0 M GdmCl, with fits to the native and unfolded subpopulations at high- and low-transfer efficiency, respectively. The peak in the shaded range corresponds to molecules without an active acceptor fluorophore. ( c ) Root mean squared end-to-end distance, r 2 1/2 , of the 39-99 segments of R15 (black) and R17 (blue) calculated from the unfolded state transfer efficiencies. ( d – f ) Representative nanosecond fluorescence correlations of donor–donor ( g DD , d ), donor–acceptor ( g DA , e ) and acceptor–acceptor ( g AA , f ) fluorescence intensities for R15 at 1.2 M GdmCl. The set of DD, DA and AA correlations for each variant and GdmCl concentration are fitted globally with a common decay rate on the 100-ns timescale, which reports on the reconfiguration of the unfolded chain (for details, see Methods ). Full size image As in the case of FRET efficiency histograms, the nsFCS experiments require a sufficient fraction of unfolded molecules to be present in the sample. However, the populations of the unfolded state at guanidinium chloride (GdmCl) concentrations far below the unfolding midpoint become too low to be detected reliably. To probe unfolded R17 even in the virtual absence of denaturant, where the conformations are most compact and internal friction is expected to be most pronounced, we employed a microfluidic device that allows millisecond mixing and was optimized for single-molecule fluorescence detection [41] , [42] ( Fig. 2 ). The denaturant is diluted rapidly by mixing GdmCl-unfolded protein with buffer solution, which enables us to populate the unfolded state transiently under native conditions. The resulting compact unfolded state can be probed by confocal single-molecule measurements in the observation channel of the device directly after mixing, where a large fraction of protein molecules are still unfolded ( Fig. 2a and b ). The unfolded subpopulation will convert to the folded state as the molecules flow down the observation channel ( Supplementary Fig. S2 ). The dynamics of the unfolded state can also be measured in the mixer: Fig. 2d–f shows examples of donor–donor, donor–acceptor and acceptor–acceptor fluorescence intensity correlation curves with a relaxation on the 100 ns timescale, typical of unfolded state dynamics [29] , [30] , [43] , [44] . The relaxation time is extracted by a global fit to all three correlations (see Supplementary Information for details). Together with the information about the distance distribution from the transfer efficiency histograms, a reconfiguration time or an effective intramolecular diffusion coefficient can be calculated [29] , [30] , [40] . In this way, unfolded state dynamics can be measured over a wide range of denaturant concentrations, and can then be used to quantify the contribution of internal friction. 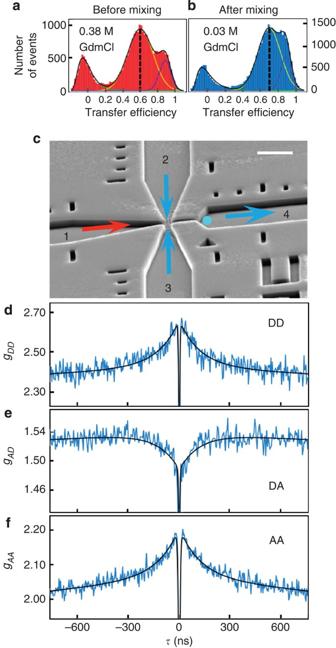Figure 2: Transient population of the unfolded state under native conditions by microfluidic mixing. (a) FRET efficiency histogram of R17 39-99 in 0.38 M GdmCl, corresponding to the conditions before mixing. (b) FRET efficiency histogram in 0.03 M GdmCl, measured in the observation region (channel 4, cyan circle) of the microfluidic device (c; scale bar, 50 μm) after dilution of the initial 0.38 M GdmCl solution (enteringviachannel 1) with native buffer appliedviachannels 2 and 3. The shift of the transfer efficiency of the unfolded state from 0.60 (a) to 0.70 (b) corresponds to the collapse of the chain on reduction in GdmCl concentration. (d–f) Nanosecond correlations of donor–donor (d, DD), donor–acceptor (e, DA) and acceptor–acceptor (f, AA) fluorescence intensities measured after mixing, fitted with a common decay rate corresponding to chain dynamics. Figure 2: Transient population of the unfolded state under native conditions by microfluidic mixing. ( a ) FRET efficiency histogram of R17 39-99 in 0.38 M GdmCl, corresponding to the conditions before mixing. ( b ) FRET efficiency histogram in 0.03 M GdmCl, measured in the observation region (channel 4, cyan circle) of the microfluidic device ( c ; scale bar, 50 μm) after dilution of the initial 0.38 M GdmCl solution (entering via channel 1) with native buffer applied via channels 2 and 3. The shift of the transfer efficiency of the unfolded state from 0.60 ( a ) to 0.70 ( b ) corresponds to the collapse of the chain on reduction in GdmCl concentration. ( d – f ) Nanosecond correlations of donor–donor ( d , DD), donor–acceptor ( e , DA) and acceptor–acceptor ( f , AA) fluorescence intensities measured after mixing, fitted with a common decay rate corresponding to chain dynamics. 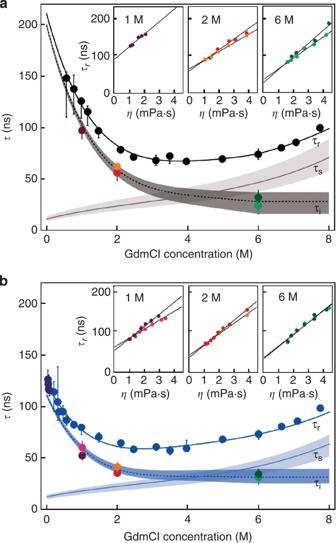Figure 3: Internal friction in unfolded spectrin domains. Dependence of the reconfiguration timesτrof the unfolded polypeptide chain on GdmCl concentration for R15 (a, black circles) and R17 (b, blue circles represent data from equilibrium experiments; dark blue circles are data from non-equilibrium experiments performed in the microfluidic mixer). Fifth-order polynomial functions were used to interpolate the values ofτr(black and dark blue solid lines). According to Eq. 1,τrcan be decomposed into a contribution corresponding to the reconfiguration time of an ideal polypeptide chain,τs(light-grey (a) and light-blue (b) solid lines), and an internal friction time,τi(dashed lines), both calculated from the value ofτiin 6 M GdmCl (see insets), and taking into account the changes in average dye-to-dye distance,r21/2(Fig. 1c), and in solvent viscosity with GdmCl concentration (seeMethods, Eq. 5). The shaded bands represent the propagation of the uncertainties in the values ofτiat 6 M GdmCl obtained from independent measurements (green circles in main graph) to the values ofτiandτs(see insets and Methods). Insets inaandbshow the dependences ofτrof unfolded R15 and R17, respectively, in 1.0, 2.0 and 6.0 M GdmCl on solvent viscosity,η, adjusted with different viscogens (glycerol: purple, yellow and dark-green circles; glucose: pink, red and light-green circles). Extrapolation ofτrtoη=0 yields the internal friction time,τl, shown in main graphs as circles color-coded as in insets. The values ofτiin 1.0 and 2.0 M GdmCl calculated in this way are in good agreement with the values calculated according to Eq. 5. Full size image Internal friction in the unfolded state of spectrin domains Figure 3 shows the reconfiguration times of unfolded R15 and R17 over the entire accessible denaturant concentration range. With the microfluidic mixing experiments, τ r for R17 could be measured down to 0.03 M GdmCl; the folding of R15 in these conditions is too fast for the unfolded state to be populated sufficiently in the mixer. For both R15 and R17, τ r ranges between 50 and 200 ns; it shows a significant increase at high GdmCl concentration due to the increasing solvent viscosity, and, more interestingly, an increase below ~2 M GdmCl. The latter observation indicates the presence of internal friction in the compact unfolded state [29] , but the similarity of the reconfiguration times of both spectrin domains shows that the slow- and fast-folding domains do not exhibit pronounced differences in internal friction in their unfolded states. Figure 3: Internal friction in unfolded spectrin domains. Dependence of the reconfiguration times τ r of the unfolded polypeptide chain on GdmCl concentration for R15 ( a , black circles) and R17 ( b , blue circles represent data from equilibrium experiments; dark blue circles are data from non-equilibrium experiments performed in the microfluidic mixer). Fifth-order polynomial functions were used to interpolate the values of τ r (black and dark blue solid lines). According to Eq. 1, τ r can be decomposed into a contribution corresponding to the reconfiguration time of an ideal polypeptide chain, τ s (light-grey ( a ) and light-blue ( b ) solid lines), and an internal friction time, τ i (dashed lines), both calculated from the value of τ i in 6 M GdmCl (see insets), and taking into account the changes in average dye-to-dye distance, r 2 1/2 ( Fig. 1c ), and in solvent viscosity with GdmCl concentration (see Methods , Eq. 5). The shaded bands represent the propagation of the uncertainties in the values of τ i at 6 M GdmCl obtained from independent measurements (green circles in main graph) to the values of τ i and τ s (see insets and Methods). Insets in a and b show the dependences of τ r of unfolded R15 and R17, respectively, in 1.0, 2.0 and 6.0 M GdmCl on solvent viscosity, η , adjusted with different viscogens (glycerol: purple, yellow and dark-green circles; glucose: pink, red and light-green circles). Extrapolation of τ r to η =0 yields the internal friction time, τ l , shown in main graphs as circles color-coded as in insets. The values of τ i in 1.0 and 2.0 M GdmCl calculated in this way are in good agreement with the values calculated according to Eq. 5. Full size image To quantify the extent of internal friction, we investigated the solvent viscosity dependence of τ r at several GdmCl concentrations ( Fig. 3 ). On extrapolation to zero solvent viscosity, we observed in all cases a value of τ r >0, confirming the presence of internal friction [5] , [6] , [15] . Surprisingly, internal friction is present even at 6 M GdmCl, where both domains are very expanded ( Fig. 1c ), and therefore the interactions within the polypeptide chains should be small. To test the possible influence of the specific viscogen used, both glycerol and glucose were employed. The good agreement of the values for τ r extrapolated to zero solvent viscosity ( Fig. 3 , insets) indicates the absence of specific interactions between protein and viscogen that might affect the results. Note also that transfer efficiency histograms provide a sensitive way of verifying that the distance distributions and thus the energetics of interactions within the unfolded states are independent of the viscogen concentration (see Supplementary Fig. S3 ), that is, the observed changes in τ r are not due to changes in unfolded state dimensions. Can we employ these results to estimate the magnitude of internal friction in the unfolded state over the entire range of GdmCl concentrations? According to a commonly used relation from polymer dynamics, which can be derived rigorously in the framework of simple models, such as the Rouse model with internal friction [45] , [46] , [47] , the overall reconfiguration time of the unfolded chain, τ r , results from the additive contributions of τ s , the reconfiguration time in the absence of internal friction, and τ i , a relaxation time due to internal friction processes. The common assumption that only the dynamics corresponding to τ s depend on solvent viscosity, η , whereas τ i does not [45] , [46] , [47] , leads to the relation where η 0 is the viscosity of the solvent in the absence of viscogen [44] . If we take into account the linear scaling of τ s with the mean squared end-to-end distance, r 2 , of the chain segment, we obtain τ s η r 2 (in this case, we assume the scaling expected for a Rouse chain, but other common models of polymer dynamics, for example the Zimm model, yield very similar results [44] ). The values of τ i measured via the viscosity dependences can be used as constraints for obtaining the GdmCl dependence of both τ i and τ s ( Fig. 3 ) (see Methods for details). The result shows that internal friction dominates the unfolded state dynamics of the spectrin domains at low GdmCl concentrations, but τ i remains in the range of 100–200 ns for both variants, orders of magnitude lower than the folding time. In summary, we find no pronounced difference in τ i between fast- and slow-folding spectrin domains, which indicates that the internal friction observed in the folding kinetics of the slow-folding domains is not present in the unfolded state, that is, the part of the reaction preceding the transition state region. Internal friction in the transition state region The early transition state, which is rate-limiting at low concentrations of denaturant, has been the subject of previous experiments [8] . Here we extend our investigation to the late transition state, which becomes rate-limiting at high GdmCl concentrations [8] , [48] , [49] , [50] , by taking advantage of the nonlinearity in the dependences of the logarithm of the unfolding rate constants on denaturant concentration (the chevron plots) [31] , [32] , [51] observed for R16 [48] , [49] and R17 [8] , [50] ( Fig. 4a ). Several models have been proposed to interpret such behaviour [31] , [32] , [51] . For our analysis, we assumed the presence of two sequential transition states separated by a high-energy intermediate [49] to quantify to what extent each of these transition states contributes to the kinetics of the overall folding reaction and how sensitive the two relative rates are to solvent viscosity. This approach allows us to assess the presence of internal friction separately for the two transition states (note, however, that our interpretation would also be valid in the framework of a broad energy barrier scenario [49] , [52] ). 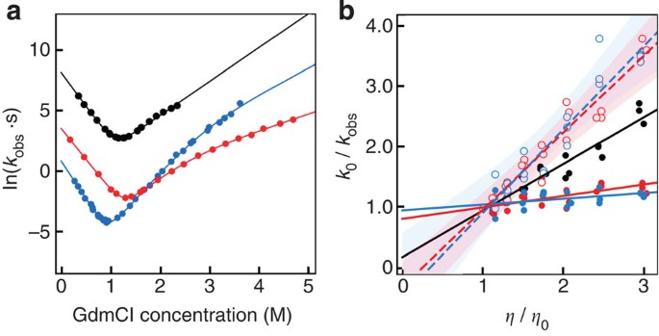Figure 4: Folding kinetics and internal friction from ensemble stopped-flow fluorescence experiments. (a) Chevron plots of R15 (black), R16 (red) and R17 (blue). R17 and R16 are fitted to a model assuming two sequential transition states and a high-energy intermediate state, whereas R15 is fitted to a two-state model with a single transition state. (b) Dependence of the reciprocal relative folding and unfolding rates on relative solvent viscosity for R15, R16 and R17 (colour code as in (a)).k0is the rate constant measured at each GdmCl concentration in the absence of viscogen;kobsis the rate measured in the presence of different amounts of viscogen;ηis the solvent viscosity; andη0is the solvent viscosity in the absence of viscogen (1.0 mPa·s). For R16 (red) and R17 (blue), the filled and empty circles represent folding over the early and late transition states, respectively. For sake of clarity, data for each domain (un)foldingviaeach transition state is presented as only one set of data with the same symbol and colour. Linear fits to these data sets are shown as solid or dashed lines for rates corresponding to the crossing of the early and late transition states, respectively. The light-red- and blue-shaded areas along the latter fits indicate confidence intervals (confidence level 90%) calculated individually for the unfolding, refolding and midpoint data sets of each domain. Figure 4: Folding kinetics and internal friction from ensemble stopped-flow fluorescence experiments. ( a ) Chevron plots of R15 (black), R16 (red) and R17 (blue). R17 and R16 are fitted to a model assuming two sequential transition states and a high-energy intermediate state, whereas R15 is fitted to a two-state model with a single transition state. ( b ) Dependence of the reciprocal relative folding and unfolding rates on relative solvent viscosity for R15, R16 and R17 (colour code as in ( a )). k 0 is the rate constant measured at each GdmCl concentration in the absence of viscogen; k obs is the rate measured in the presence of different amounts of viscogen; η is the solvent viscosity; and η 0 is the solvent viscosity in the absence of viscogen (1.0 mPa·s). For R16 (red) and R17 (blue), the filled and empty circles represent folding over the early and late transition states, respectively. For sake of clarity, data for each domain (un)folding via each transition state is presented as only one set of data with the same symbol and colour. Linear fits to these data sets are shown as solid or dashed lines for rates corresponding to the crossing of the early and late transition states, respectively. The light-red- and blue-shaded areas along the latter fits indicate confidence intervals (confidence level 90%) calculated individually for the unfolding, refolding and midpoint data sets of each domain. Full size image Figure 4b shows the dependence on solvent viscosity of the relative folding and unfolding rates of R15 and those corresponding to the early and late transition states of R16 and R17. Folding and unfolding of R16 and R17 over the early transition state show much less solvent viscosity dependence than folding and unfolding of R15 [8] . This behaviour reflects the large internal friction in the early transition state of R16 and R17. Intriguingly, the behaviour resulting from unfolding over the late transition state ( Fig. 4a ) is very different. In this case, a pronounced solvent viscosity dependence of the folding and unfolding rates is observed for both R16 and R17 ( Fig. 4b ), with a slope close to unity, as expected for a process without internal friction. The kinetics corresponding to the second transition state of R15 are not accessible by stopped-flow measurements because of the high unfolding rates at high denaturant concentrations. However, considering the fast folding of R15, the linear dependence of its folding and unfolding rates on solvent viscosity, and the mechanistic interpretation suggested on the basis of extensive protein-engineering experiments [53] , it is very unlikely for internal friction to develop in the context of a hypothetical late transition state. This surprising result clearly indicates that only the early, less native-like, transition states of R16 and R17 show indications for the presence of internal friction; in the second transition states, internal friction is undetectably low. In a next step, can we go beyond such a qualitative statement and compare internal friction at the different stages of the folding reaction more quantitatively? Internal friction along the folding reaction A common feature of the viscosity dependencies of both the reconfiguration times in the unfolded state and the folding and unfolding times of the spectrin domains is the existence of a non-zero intercept with the relaxation time axis on extrapolation to η =0. This behaviour is the characteristic signature of friction within the protein that is largely independent of solvent viscosity [15] , [45] . For the unfolded state, the overall relaxation time of the chain is well described by equation (1), as expected from polymer theory [45] , [46] , [47] . For the folding dynamics, we use a modified Kramers-type picture originally suggested by Ansari et al . [15] in the context of conformational changes in folded proteins. This model assumes that the contribution of friction from collisions, with the solvent on the one hand and other atoms within the protein on the other, results in an additivity of external (that is, solvent-mediated) and internal (that is, protein-mediated) viscosities, η and σ , respectively. The resulting expression for the folding time, τ f (the inverse folding rate coefficient), is where σ TS is the value of σ in the transition state region [26] , [54] ; C contains all contributions to the preexponential factor except η and σ TS ; Δ is the height of the free energy barrier; k B is the Boltzmann constant and T is temperature. In analogy to equation (1), τ f can be considered a sum of a solvent viscosity-dependent relaxation time, τ fs , and a solvent viscosity-independent relaxation time, τ fi , which would equal zero in the absence of internal friction. An analogous expression is valid for the unfolding time, τ u . Assuming that the variation of solvent viscosity does not change the equilibrium constant of the reaction (note that the equilibrium denaturation free energy is kept constant here by the addition of GdmCl), σ TS is expected to be the same for folding and unfolding kinetics. Because of microscopic reversibility, the extrapolation of the folding and unfolding times, respectively, to η =0 should thus yield the same value of σ TS , that is, the contribution of internal viscosity at the transition state should be independent of the direction of barrier crossing. The viscosity dependences of the folding and unfolding rates observed experimentally ( Fig. 5 ) for R15, R16 and R17 are in good agreement with this prediction ( Fig. 5 ). Note that for Δ→0, that is, in the absence of a free energy barrier, equation (2) converges to equation (1), indicating the consistency of equation (1) for unfolded state dynamics with equation (2) for diffusive barrier crossing. Note also that a non-additive contribution of internal friction (or internal viscosity, equation (2)) to the relaxation dynamics of the system [55] would always lead to an overall relaxation time of zero when extrapolated to zero solvent viscosity and is thus not considered here. Likewise, in view of the close structural similarity of the spectrin domains, generic solvent properties [56] are unlikely to cause the pronounced differences in experimentally observed internal friction ( Fig. 3 ) [8] . 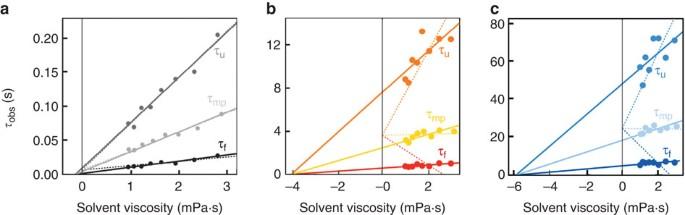Figure 5: The solvent viscosity dependence of the folding kinetics is well described by diffusive barrier crossing. (a–c) Solvent viscosity dependences of the folding and unfolding times of R15 (a), R16 (b) and R17 (c) corresponding to crossing of the early transition state at ΔG=1.5 kcal mol−1(τu,τf) and at ΔG=0 (τmp). Global fits according to equation (2), with a common value of internal viscosity at the transition state,σTS(solid lines), describe the data well, in contrast to global fits according to equation (1), with a common value of an internal friction time (dotted lines), which supports the applicability of equation (2) for folding dynamics. The resulting values ofσTSare (0.14±0.08), (3.8±1.0) and (5.6±2.0) mPa s for R15, R16 and R17, respectively. Figure 5: The solvent viscosity dependence of the folding kinetics is well described by diffusive barrier crossing. ( a – c ) Solvent viscosity dependences of the folding and unfolding times of R15 ( a ), R16 ( b ) and R17 ( c ) corresponding to crossing of the early transition state at Δ G =1.5 kcal mol −1 ( τ u , τ f ) and at Δ G =0 ( τ mp ). Global fits according to equation (2), with a common value of internal viscosity at the transition state, σ TS (solid lines), describe the data well, in contrast to global fits according to equation (1), with a common value of an internal friction time (dotted lines), which supports the applicability of equation (2) for folding dynamics. The resulting values of σ TS are (0.14±0.08), (3.8±1.0) and (5.6±2.0) mPa s for R15, R16 and R17, respectively. Full size image Based on equation (2) and Fig. 4b , we can compare the values of τ fi corresponding to the early and late transition states of the different spectrin variants ( Fig. 6 ). We obtain values for τ fi of (95±11) and (7.3±0.5) ms for the early transition states of R17 and R16, respectively, but only (0.016±0.009) ms for R15, which in part reflects the difference in internal friction between the slow- and fast-folding spectrin domains. For the late transition state, we can only estimate upper bounds for τ fi because the underlying internal friction is too low to influence the overall kinetics to a detectable degree; we obtain 28 and 10 μs for R17 and R16, respectively (see Methods for details). For comparison, the values of τ i in the unfolded states of R17 and R15 under native conditions are only about 110 and 200 ns, respectively. For the rate-limiting early transition states of R15, R16 and R17, we obtain values for σ TS of (0.14±0.08), (3.8±1.0) and (5.6±2.0) mPa s, respectively ( Fig. 5 , Supplementary Table S1 ). According to equation (2), we expect the folding and unfolding times to be increased compared with the case without internal friction (but assuming the same values of Δ and C ) by ( σ TS + η )/ η , that is, by factors of approximately 5 and 7 for R16 and R17, respectively, ( Supplementary Table S1 ). Remarkably, the relaxation rates of R15 and the recently identified E18F/K25V variant of R16, which folds and unfolds 40-fold faster than wild-type R16 but has an unchanged value of σ TS , differ by about this factor of five [57] . This agreement supports the hypothesis that the 40-fold increase in rate for the variant is caused by a decrease in barrier height, but the remaining difference in rates between R15 and R16 E18F/K25V is caused by the difference in σ TS , that is, in internal friction [57] . 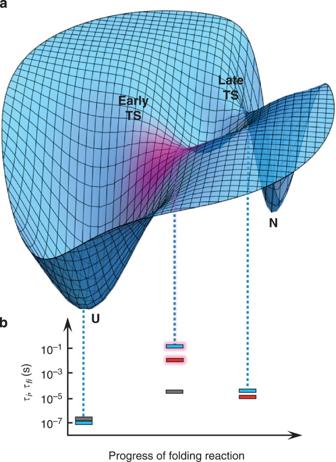Figure 6: Internal friction is localized in the early transition state (TS) of spectrin domain folding. (a) Cartoon of the folding free energy surface of the spectrin domains illustrating the localization of internal friction at the early TS of R16 and R17 (magenta). The dotted lines indicate the regions of the energy landscape corresponding to the solvent viscosity-independent time constants (b) at the different stages of the folding reaction (τiin the unfolded state, see equation (1);τfiat the TS, see equation (2)) for R15 (black), R16 (red) and R17 (blue). The folding dynamics are most affected by internal friction at the early TS, whereτfifor R16 and R17 has a magnitude comparable to the folding time (magenta-shaded bars). The corresponding deceleration of folding dynamics by internal friction is about 5-fold for R16 and about 7-fold for R17 (Supplementary Table S1). Note that the presence of a late TS is uncertain for R15 because of its high folding rates, which make the kinetic data inaccessible by stopped flow at high GdmCl concentrations (cf.Fig. 4a). Figure 6: Internal friction is localized in the early transition state (TS) of spectrin domain folding. ( a ) Cartoon of the folding free energy surface of the spectrin domains illustrating the localization of internal friction at the early TS of R16 and R17 (magenta). The dotted lines indicate the regions of the energy landscape corresponding to the solvent viscosity-independent time constants ( b ) at the different stages of the folding reaction ( τ i in the unfolded state, see equation (1); τ fi at the TS, see equation (2)) for R15 (black), R16 (red) and R17 (blue). The folding dynamics are most affected by internal friction at the early TS, where τ fi for R16 and R17 has a magnitude comparable to the folding time (magenta-shaded bars). The corresponding deceleration of folding dynamics by internal friction is about 5-fold for R16 and about 7-fold for R17 ( Supplementary Table S1 ). Note that the presence of a late TS is uncertain for R15 because of its high folding rates, which make the kinetic data inaccessible by stopped flow at high GdmCl concentrations (cf. Fig. 4a ). Full size image We find that the marked effects of internal friction on the folding and unfolding rates of R16 and R17 are present only in the early transition state; in the late transition state, internal friction remains undetectable; in the compact unfolded states of both slow- and fast-folding spectrin domains, even though they show a pronounced influence of internal friction on their reconfiguration dynamics, the internal friction times are in the sub-microsecond range, orders of magnitude too low for having a measurable effect on the millisecond folding times. The effect of internal friction on the free energy surface of the spectrin domains thus seems to be far from evenly distributed along the reaction; instead, it is highly localized to the early transition state ( Fig. 6 ). This finding is surprising, given the reasonable assumption that internal friction should increase monotonically with the number of interactions within a polypeptide chain, which would imply that it should increase on moving from the early to the late transition state. Such a scenario, which assumes that internal friction results from averaging over rather uniform properties of the polypeptide chain, and describes, for example, the behaviour we observe in the unfolded state ( Fig. 3 ) [29] , [44] , does not seem to apply to the barrier-crossing process. Instead, our results are more consistent with a group of rather specific interactions that need to be correctly established during passage of the early transition state, in keeping with a nucleation-type mechanism [58] . Additional support for this interpretation comes from the results of extensive protein-engineering experiments [53] , which show that changing only five amino acids in a key region of the A helix is sufficient to increase the folding and unfolding rates of the slow folders R16 and R17 into the same range as the much faster-folding R15 and to greatly reduce the influence of internal friction. The Φ-value analysis of the corresponding variants is indicative of a concomitant change in folding mechanism, from a diffusion–collision-type in R16 and R17 to the nucleation–condensation-type reaction characteristic of R15. This seems to confirm the hypothesis that the origin of the internal friction that leads to the insensitivity to solvent viscosity observed for R16 and R17 may lie in the search for the correct register in the packing of preformed helices [8] , [53] . The low solvent viscosity dependence would indicate, however, that only small-amplitude motions against the solvent are involved. What do these findings implicate for a theoretical description of protein-folding dynamics? In the simplest one-dimensional diffusive model based on Kramers theory [54] , the rate of barrier crossing, k f , is given by where ω U and ω TS characterize the curvatures of the potential in the unfolded well and on top of the barrier (that is, in the transition state region), respectively, and D TS is the effective diffusion coefficient in the barrier region. In the case of experiments based on single-molecule FRET or force spectroscopy, for instance, the reaction coordinate would correspond to an intramolecular distance, and the corresponding shape and diffusion parameters are starting to become available from optical and force-based single-molecule experiments [29] , [36] , [39] , [44] , [59] . For the spectrin domains, where the results suggest that interactions between a few residues have a key role for internal friction in folding kinetics, it is plausible that a relatively small change in the number of contacts, resulting from conformational rearrangements involved in crossing the transition state barrier, could give rise to a comparatively large change in free energy. In the Kramers-type picture (equation (3)), such behaviour would correspond to a larger curvature of the free energy surface at the transition state compared with that for unfolded state, resulting in a substantial difference between ω TS and ω U [23] . The results shown in Fig. 5 suggest that a diffusive description of the folding dynamics is applicable, in spite of the importance of highly specific interactions at the transition state. A promising strategy for testing the importance of internal friction on the dynamics in the transition state region and the applicability of a diffusive description for the folding of spectrin domains might be measurements of transition path times, which are starting to become accessible in single-molecule experiments [3] ; for folding reactions involving internal friction, the transition path time should be longer by a factor of approximately ( σ TS + η )/ η compared with the reaction without internal friction [3] . We hope that the increasing amount of detail available from experimental results like ours will stimulate simulations and the development of quantitative theoretical concepts that go beyond the simple one-dimensional picture used here, and will allow us to better describe the complexity of folding dynamics and understand the role and mechanisms of internal friction. Preparation and labelling of proteins The labelling sites were selected to minimize the effects on the conformational stability and folding mechanism, based on the extensive previous protein-engineering studies [48] , [50] . The separations of the dyes in the sequence and the folded structure were chosen such that (a) the transfer efficiencies expected in the unfolded state would be in a range resulting in good sensitivity for the determination of intramolecular distance distributions and dynamics, and that (b) a pronounced separation of folded and unfolded subpopulations in FRET efficiency histograms could be achieved. For labelling of the spectrin domains, cysteine residues were introduced by site-directed mutagenesis at positions 39 and 99, and the proteins were expressed and purified as described previously [60] . In R17, an endogenous cysteine at position 68 was exchanged to alanine to avoid multiple labelling. For labelling, a 1.3:1 molar excess of reduced protein was incubated with Alexa Fluor 488 maleimide (Invitrogen) at 4 °C for ~10 h. Unreacted dye was removed by gel filtration (G25 desalting; GE Healthcare Biosciences AB, Uppsala, Sweden), and the protein was incubated with Alexa Fluor 594 maleimide at room temperature for ~2 h. Differently labelled variants were separated by ion-exchange chromatography (MonoQ HR 5/5; GE Healthcare Biosciences AB). Ensemble folding and unfolding kinetics of R15, R16 and R17 were monitored by the change in tryptophan fluorescence on an SX20 stopped-flow spectrometer (Applied Photophysics) and fitted as described previously [8] . Briefly, chevron plots for R15 were fitted to a two-state model and those for R16 and R17 to a sequential transition state model [31] as described in detail by Scott and Clarke [49] . The calculation of folding and unfolding times (τ f and τ u ) at Δ G =1.5 kcal mol −1 and of the relaxation time τ mp at Δ G =0 has previously been described for the first transition state [8] . Those for the second transition state were calculated in an analogous manner using the fitted second transition state parameters. Single-molecule fluorescence spectroscopy Measurements were performed using both a custom-built confocal microscope and a MicroTime 200 confocal microscope equipped with a HydraHarp 400 counting module (PicoQuant, Berlin, Germany). The donor dye was excited with a diode laser at 485 nm (dual mode: continuous wave and pulsed; LDH-D-C-485, PicoQuant) at an average power of 100 μW at the sample. Single-molecule FRET efficiency histograms were acquired in samples with a protein concentration of about 20–50 pM, with the laser in either continuous-wave mode or pulsed mode at a repetition rate of 64 MHz; photon counts were recorded with a resolution of 16 ps at the counting electronics (time resolution was thus limited by the timing jitter of the detectors). The nsFCS measurements were performed in samples with a protein concentration of ~1 nM, over a period of 16 h, at an average power of 70 μW with the laser in continuous-wave mode. For rapid mixing experiments, microfluidic mixers fabricated by replica moudling in polydimethylsiloxane (PDMS) were used as described previously [41] , [42] . The experiments were performed with pressures of 13.8 kPa (2.0 psi) applied to the side channels (no. 3 and 4 in Fig. 2c ) and 6.9 kPa (1.0 psi) to the middle channel. The flow stability was monitored by analysing the time evolution of the fluorescence intensity cross-correlation. The nsFCS measurements in the mixer were performed over a period of 2–10 h and analysed as detailed below (‘ nsFCS measurements ’). Controls of the contribution of dye quenching to the acceptor autocorrelation were carried out with a continuous wave HeNe laser (594 nm; CVI Melles Griot, Albuquerque, NM, USA) at a power of 16 μW at the sample. All measurements were performed in 50 mM sodium phosphate buffer, pH 7.0, 140 mM β-mercaptoethanol (Sigma), 20mM cysteamine hydrochloride (Sigma) and 0.001% Tween 20 (Pierce) with varying concentrations of GdmCl (Pierce). Tween 20 was used to prevent surface adhesion of the proteins, and the photoprotective agents β-mercaptoethanol and cysteamine hydrochloride were employed to minimize chromophore damage and enhance brightness. For experiments in the microfluidic device, the Tween 20 concentration was increased to 0.01%. Guanidine concentrations were measured with an Abbe refractometer (Krüss, Germany), and viscosities of the solutions were measured with a digital viscometer (DV-I+; Brookfield Engineering, Middleboro, MA, USA) with a CP40 spindle at 30 or 60 r.p.m., which allows determination of viscosity with an uncertainty of 0.05–0.1 mPa·s. nsFCS measurements Fluorescence intensities of donor and acceptor fluorophores were recorded with a four-channel HydraHarp 400 Picosecond Event Timer (PicoQuant) and correlated with a binning time of 1 ns. To avoid effects of detector dead times and afterpulsing on the correlation functions, the signal was recorded with two detectors each for donor and acceptor and cross-correlated between detectors. Auto- and cross-correlation curves were fitted over a time window of 2.5 μs with where i and j correspond to donor or acceptor fluorescence emission, N is the effective mean number of molecules in the confocal volume, c ab , τ ab , c cd and τ cd are the amplitudes and time constants of the antibunching and chain dynamics, respectively [29] , [30] , whereas c T and τ T refer to the triplet blinking of the fluorophores. The three correlation curves were fitted globally with the same values of τ cd and a fixed value of τ T estimated from the fit of the whole acceptor–acceptor autocorrelation curve from nanoseconds to seconds. The amplitude and the lifetime of the antibunching and the triplet amplitude were fit with a free independent decay component for each correlation curve. The errors associated with the global fit were estimated by resampling the experimental dataset via a bootstrap method. Viscosity dependence of τ r The reconfiguration times τ r measured as a function of viscosity at different GdmCl concentrations ( Fig. 3 insets) were fitted to a linear function, yielding the reconfiguration time at 0 M GdmCl, which corresponds to the τ i , that is, the internal friction contribution, at every set of conditions. To quantify the contribution of internal friction to the observed reconfiguration time, we subtract τ i (6 M), the average of the two values obtained for the internal friction time in 6 M GdmCl with the two viscogens, from the value of the reconfiguration time calculated at the same GdmCl concentration, τ r (6 M). The resulting time, τ s (6 M), represents the reconfiguration time of an ideal polypeptide chain in the absence of internal friction. τ s depends on both the polypeptide chain dimensions and the solvent viscosity, therefore its value can be calculated at any GdmCl concentration, provided that the dimension of the chains are known, according to: where η is the solvent viscosity, and and are the GdmCl-dependent dye-to-dye distance and the dye-to-dye distance at 6 M GdmCl, respectively, obtained from the transfer efficiency histograms. The value of τ i is then calculated at all GdmCl concentrations by subtracting τ s from τ r . Because the quantification of τ i and τ s relies on the value of τ i at 6 M GdmCl, an estimation of the error associated with these quantities can be obtained by propagating the uncertainty of τ i (6 M). The s.d. of τ i (6 M) is calculated from the values of τ i extrapolated at η =0 from the viscosity-dependent experiment carried out with glycerol and glucose. In Fig. 3 , the grey- and blue-shaded areas for τ i and τ s are calculated with equation (5), assuming a distribution of τ i (6 M) within one s.d. Calculation of friction parameters for the transition states From the definition of σ at the transition state (equation (2) and Supplementary Fig. S5 ), where τ f ( η =0) is the folding time extrapolated to zero solvent viscosity, and τ fs is the solvent-dependent contribution to the folding time, calculated as τ f − τ fi , where τ fi is the solvent-independent internal friction time. Given that the value of σ seems to be invariant with GdmCl concentration (‘ Internal friction along the folding reaction ’ in main text), we calculate σ for the early transition state from a global fit of refolding, unfolding and midpoint kinetics ( Fig. 5 ). τ fi can then be calculated for any denaturant concentration from Individual and global linear fits of the three data sets corresponding to refolding, unfolding and midpoint kinetics over the late transition state in R16 and R17 ( Fig. 4 ) extrapolate to small negative values on the τ obs axis ( Supplementary Fig. S4 , corresponding to small negative values on the k 0 / k obs axis of Fig. 4b ). Instead of just assuming that internal friction is negligible within experimental error for these processes, we calculated confidence intervals (confidence level of 90%) for the individual fits of each of these three data sets for each domain and used the average of the highest values within these confidence intervals to estimate an upper bound on σ within experimental uncertainty ( Supplementary Fig. S4 ). The maximum σ values were then used to calculate an upper bound for the expected internal friction times for the two domains according to equation (7) ( Supplementary Table S1 ). How to cite this article: Borgia, A. et al . Localizing internal friction along the reaction coordinate of protein folding by combining ensemble and single-molecule fluorescence spectroscopy. Nat. Commun. 3:1195 doi: 10.1038/ncomms2204 (2012).